Broadband graphene terahertz modulators enabled by intraband transitions Terahertz technology promises myriad applications including imaging, spectroscopy and communications. However, one major bottleneck at present for advancing this field is the lack of efficient devices to manipulate the terahertz electromagnetic waves. Here we demonstrate that exceptionally efficient broadband modulation of terahertz waves at room temperature can be realized using graphene with extremely low intrinsic signal attenuation. We experimentally achieved more than 2.5 times superior modulation than prior broadband intensity modulators, which is also the first demonstrated graphene-based device enabled solely by intraband transitions. The unique advantages of graphene in comparison to conventional semiconductors are the ease of integration and the extraordinary transport properties of holes, which are as good as those of electrons owing to the symmetric conical band structure of graphene. Given recent progress in graphene-based terahertz emitters and detectors, graphene may offer some interesting solutions for terahertz technologies. Graphene, a two-dimensional semiconductor with zero bandgap, has attracted much attention for its extraordinary carrier transport properties [1] , leading to impressive device performance [2] ; its optoelectronic properties are equally noteworthy. On the basis of their peculiar band structures, single-layer graphene and Bernal-stacked bilayer graphene have been proposed for novel terahertz [3] , [4] , [5] , [6] , [7] and optoelectronic devices [8] , with some successful experimental demonstrations [9] , [10] , [11] , [12] . Interband and intraband transitions under optical excitation in graphene have been investigated by various groups [13] , [14] , [15] , [16] , [17] , [18] , [19] . Thus far, all the experimental studies confirmed the following theoretical expectations. First, interband transitions dominate in the infrared/visible range, resulting in a constant absorption of ~2.3% by single-layer graphene at normal incidence and modulation of infrared absorption from ~2.3 to ~0% by electrically tuning its Fermi level. Second, intraband transitions dominate in the terahertz range, resulting in an optical conductivity well described by the Drude model. Plasmonic effects in graphene were also recently observed [7] , which are important in the transition range from terahertz to infrared. Rooted in these understandings, several devices based on interband transitions have been demonstrated, including transparent electrodes [10] , photodetectors [11] , and broadband infrared electro-optical modulators [12] . However, to date, device applications of graphene optical properties in the terahertz range remain largely unexplored. Lying between radio frequency and infrared, terahertz electromagnetic waves have been notoriously difficult to produce, modulate and detect. Recent progress in sources and detectors is turning what was only recently called the 'terahertz gap' into one of the most rapidly growing technological fields [20] , [21] , [22] . At present, high-performance elements to control and manipulate terahertz electromagnetic waves, such as modulators and active filters, are in high demand to develop sophisticated communication and imaging systems. However, terahertz wave modulators studied to date generally exhibit compromised performance between modulation depth, broadband operation, signal attenuation, polarization dependence, on-chip integrability and structural complexity [23] , [24] , [25] , [26] . We have recently proposed a novel room-temperature broadband terahertz intensity modulator using graphene, which is capable of avoiding these trade-offs [27] . By tuning the Fermi level in graphene, we tune the density of states available for intraband transitions under terahertz illumination and therefore terahertz transmission. Graphene supports a high carrier concentration (up to 1×10 14 cm −2 ) [28] as well as outstanding carrier mobility (>20,000 cm 2 V −1 s −1 for n s ~5×10 12 cm −2 ) [29] for both holes and electrons owing to its symmetric conical band structure, which leads to a good tunable conductivity range and a high maximum hole/electron conductivity comparable to that of conventional epitaxial semiconductors achievable only by electrons. Our theoretical calculations [27] show that transmission can be modulated between nearly zero and unity by a single-layer graphene over a broad range of carrier frequencies up to a few terahertz, which is in sharp contrast with its absorption of 2.3% in the infrared/visible range. Simultaneously, extremely low signal attenuation at room temperature, induced by the intrinsic device (<0.2 dB per graphene layer), can be realized by taking advantage of its reasonably low minimum conductivity, when the Fermi level is tuned at its Dirac point. Here we present the first experimental demonstration of this type of device, which consists of a single-layer graphene-based prototype exhibiting an intensity modulation depth of 15% and a modulation frequency of 20 kHz, using a 570-GHz carrier at room temperature. Even though its modulation depth is limited by the quality of graphene used and the modulation speed by the large device size, the result of this work represents a significant improvement over the previously reported inherently broadband devices based on AlGaAs/GaAs structures [25] , [26] , which showed a maximum intensity modulation depth of 6%. An impressive and flat modulation amplitude was reported over a wide frequency range in a metamaterial-based device [30] when taking into account contributions from both amplitude and phase of the electric field employing a field-resolved detection scheme. However, these metamaterial devices are inherently narrowband in terms of amplitude/phase modulation. The active tuning of terahertz transmission demonstrated in this work suggests that graphene-based structures are attractive for terahertz modulators and electrically reconfigurable filters and attenuators. Free from lattice-matching often required in epitaxial semiconductor heterostructures, these graphene modulators may be easily integrated with existing solid-state continuous wave (CW) terahertz sources such as quantum cascade lasers [31] and resonant tunnelling diode oscillators [32] , and with terahertz detectors such as Schottky diodes [33] and backward diodes [34] , or future graphene-based terahertz emitters and detectors [3] , [4] , [5] . The possibilities of facile integration make graphene modulators promising as single-chip solutions for compact and cost-effective transceivers in the terahertz band. Operating principle and modulator structures Optical absorption in graphene involves two processes: carrier intraband transitions and interband transitions ( Fig. 1a ), which can be expressed using the optical conductivity σ ( ω ): σ ( ω )= σ intra ( ω )+ σ inter ( ω ), where ω is the angular frequency of the photon. Calculations of optical conductivity have shown that, for short wavelengths (that is, infrared and visible range), the graphene optical conductivity is determined by interband transitions, whereas, for long wavelengths (that is, terahertz range), it is dominated by intraband transitions [13] , [14] , [19] . In the visible and infrared range, where interband transitions dominate, the graphene optical conductivity is nearly independent of the Fermi energy in graphene ( E F ) and the optical frequency ( hv ), as long as hv>2E F ; a classical value of optical conductivity (dynamic) σ ( ω )= e 2 /4ħ gives rise to a constant absorption of 2.3% by single-layer graphene [15] . The combination of the exceptional transport properties of graphene and its transparency in the visible range has led to demonstration of transparent electrodes employing graphene [10] . By electrically tuning the Fermi level in graphene, interband transitions at hv =2 E F can be turned on and off [17] , [18] , leading to the recent demonstration of broadband infrared modulators [12] . Because modulation by single-layer graphene, in this frequency range, is only ~2.3% at normal incidence, a waveguide platform was adopted [12] . On the other hand, in the terahertz range where intraband transitions dominate, graphene behaves like a conductive film, and its optical conductivity closely follows its electrical conductivity. Optical conductivity can be described by a simple Drude model of the form [13] , [14] , [19] σ ( ω )= σ DC ( E F )/(1+ ω 2 τ 2 ), where σ DC ( E F ) represents the DC electrical conductivity and τ is the carrier momentum scattering time. As suggested by this equation, terahertz absorption in graphene can be modulated by tuning its electrical conductivity or Fermi level; when ωτ· 1, σ ( ω )~ σ DC ( E F ); when ωτ >1, σ ( ω ) < σ DC ( E F ). 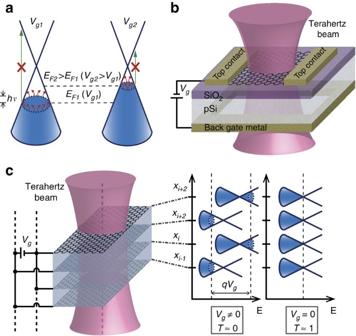Figure 1: Operating principle and modulator structures. (a) Conical band structure of graphene and optical processes in graphene. Intraband transitions (red arrows) dominate under terahertz illumination where the photon energy (h•) is generally smaller than 12.4 meV (3 THz); when tuning the Fermi level in graphene (EF), using a voltageVg, one can tune the density of states available for intraband transitions, thus terahertz transmission. Interband transitions (green arrows) from valence to conduction band dominate in the infrared/visible range. (b) Schematic of the proof-of-concept graphene terahertz modulator. The single-layer graphene was prepared on a SiO2/p-Si substrate. The top contacts were used to monitor the graphene conductivity, and the bottom ring-shaped gate was used to tune the graphene Fermi level, that is, conductivity. Terahertz transmission spectroscopy and mapping were performed in the 570–630-GHz frequency band. The device size is ~1.5 cm×1.5 cm. All measurements were carried out at 300 K. (c) Schematic of the proposed terahertz modulator, comprised of stacked graphene pairs with capacitively coupled 2DHG in the valence band and 2DEG in the conduction band, to overcome potentially limited modulation by a single-layer graphene. Also shown are the energy-band diagrams of two graphene pairs in the middle of the stack (xjstands for the vertical position of thejth graphene layer). At zero bias (Vg=0 V), the Fermi level is at the Dirac point for all graphene layers, resulting in near-unity terahertz transmission (T). With an applied bias, the Fermi level moves into the valence and conduction band in the graphene pair, leading to near-zero terahertz transmission. Figure 1: Operating principle and modulator structures. ( a ) Conical band structure of graphene and optical processes in graphene. Intraband transitions (red arrows) dominate under terahertz illumination where the photon energy ( h • ) is generally smaller than 12.4 meV (3 THz); when tuning the Fermi level in graphene ( E F ), using a voltage V g , one can tune the density of states available for intraband transitions, thus terahertz transmission. Interband transitions (green arrows) from valence to conduction band dominate in the infrared/visible range. ( b ) Schematic of the proof-of-concept graphene terahertz modulator. The single-layer graphene was prepared on a SiO 2 / p -Si substrate. The top contacts were used to monitor the graphene conductivity, and the bottom ring-shaped gate was used to tune the graphene Fermi level, that is, conductivity. Terahertz transmission spectroscopy and mapping were performed in the 570–630-GHz frequency band. The device size is ~1.5 cm×1.5 cm. All measurements were carried out at 300 K. ( c ) Schematic of the proposed terahertz modulator, comprised of stacked graphene pairs with capacitively coupled 2DHG in the valence band and 2DEG in the conduction band, to overcome potentially limited modulation by a single-layer graphene. Also shown are the energy-band diagrams of two graphene pairs in the middle of the stack ( x j stands for the vertical position of the j th graphene layer). At zero bias ( V g =0 V), the Fermi level is at the Dirac point for all graphene layers, resulting in near-unity terahertz transmission ( T ). With an applied bias, the Fermi level moves into the valence and conduction band in the graphene pair, leading to near-zero terahertz transmission. Full size image The active device can consist of one ( Fig. 1b ) or multiple ( Fig. 1c ) capacitively coupled graphene-semiconductor or graphene–graphene pairs, so that holes are induced in one layer whereas electrons are induced in the second layer [27] . At zero bias, the Fermi level is at the Dirac point of all graphene layers, thus introducing minimum insertion loss or signal attenuation. When a bias is applied, two-dimensional hole gases (2DHGs) are induced in the graphene layers connected to the positive power supply and two-dimensional electron gases (2DEGs) in the other graphene layers connected to the negative power supply. Besides facile integration with other material platforms, another unique advantage of graphene over the conventional semiconductors lies in its excellent hole-transport properties. Since hole and electron mobilities and their density of states are the same due to the graphene symmetric band structure, each graphene layer can contribute equally to terahertz modulation. The stacked structure can help overcome the potentially limited modulation in a single graphene layer realizable in experiments. To demonstrate the potential of graphene for terahertz modulation, we fabricated a proof-of-concept terahertz modulator, using a single-layer graphene of about 1.5 cm×1.5 cm on top of SiO 2 / p -Si substrate with two top contacts to graphene and one bottom ring gate contact ( Fig. 1b ). The p -type Si substrate with a doping concentration of ~1×10 15 cm −3 was selected to facilitate terahertz direct detection by avoiding severe attenuation of terahertz beams in a highly conductive substrate. 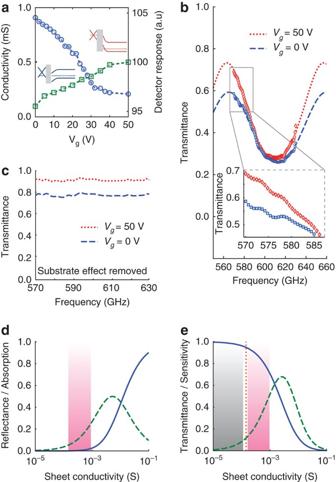Figure 2: Measured and modelled static characteristics. (a) Measured DC conductivity of graphene (blue circles) and detector response (green squares) at 600 GHz as a function of the back gate voltage (Vg). The inset shows energy-band diagrams of the graphene/SiO2/p-Si device. At 0 V, the Fermi levelEFin graphene is ~380 meV below the Dirac point, andp-Si substrate is under depletion46; at 50 V,EFin graphene is near the Dirac point and a 2D hole gas in Si accumulates near the SiO2/Si interface. (b) Measured (symbols) and modelled (lines) intensity transmittance as a function of frequency for back gate voltages of 0 V (blue) and 50 V (red). The inset is the close-up of transmittance near 570 GHz showing a maximum modulation of 15±2% at 570 GHz. (c) Transmittance after subtracting both the cavity effect and free carrier absorption due to the lightly doped bulkp-Si substrate. (d) Modelled absorption (green dashed line) and reflectance (blue solid line) as a function of graphene optical conductivity. The pink-shaded area indicates the range of graphene DC conductivity observed in this study. (e) Modelled intensity transmittance as a function of graphene optical conductivity (blue solid line) and the associated transmission sensitivity (green-dashed line), defined as the derivative of transmittance with respect to the logarithm of conductivity. Also marked on the graph are a typical minimum DC conductivity of graphene,4e2/h~0.15 mS (orange line), and the range of Si 2D hole gas DC conductivity (grey shaded area). Static characteristics Figure 2a shows the measured intensity transmittance at 600 GHz and the graphene DC conductivity as a function of the back gate voltage from 0 to 50 V. As expected, the transmittance increases with decreasing DC electrical conductivity of graphene. The graphene is p -type in the entire range of the gate voltage swing because its minimum conductivity or Dirac point occurs at V g ≥50 V. Figure 2b presents the experimental intensity transmittance as a function of frequency at V g =0 and 50 V. The maximum transmittance change (that is, modulation depth), defined as |( T (50V)− T (0V))/ T (50V)|, was calculated to be 15±2% at 570 GHz. Also shown in Fig. 2b is the calculated transmittance using a Si substrate with a thickness of 480 μm and a constant bulk conductivity of 40 mS cm −1 , and graphene conductivity of 0.9 mS at 0 V and 0.2 mS at 50 V. The excellent agreement between the measured and simulated results, using experimentally determined parameters, indicates that terahertz transmission in graphene can indeed be described by the aforementioned Drude model in this frequency range, and that the voltage-dependent free carrier absorption in the Si substrate does not have a significant role in the observed terahertz modulation, which we discuss in more details in the Methods. It is also worth noting that the peak transmittance of the two curves does not occur at the same frequency, that is, a small phase shift, which most likely stems from the simplified assumptions adopted in the model. The maximum transmission lower than unity is primarilydue to free carrier absorption in the bulk p -Si, and the oscillatory behaviour is due to Fabry–Perot interference. Figure 2: Measured and modelled static characteristics. ( a ) Measured DC conductivity of graphene (blue circles) and detector response (green squares) at 600 GHz as a function of the back gate voltage ( V g ). The inset shows energy-band diagrams of the graphene/SiO 2 / p -Si device. At 0 V, the Fermi level E F in graphene is ~380 meV below the Dirac point, and p -Si substrate is under depletion [46] ; at 50 V, E F in graphene is near the Dirac point and a 2D hole gas in Si accumulates near the SiO 2 /Si interface. ( b ) Measured (symbols) and modelled (lines) intensity transmittance as a function of frequency for back gate voltages of 0 V (blue) and 50 V (red). The inset is the close-up of transmittance near 570 GHz showing a maximum modulation of 15±2% at 570 GHz. ( c ) Transmittance after subtracting both the cavity effect and free carrier absorption due to the lightly doped bulk p -Si substrate. ( d ) Modelled absorption (green dashed line) and reflectance (blue solid line) as a function of graphene optical conductivity. The pink-shaded area indicates the range of graphene DC conductivity observed in this study. ( e ) Modelled intensity transmittance as a function of graphene optical conductivity (blue solid line) and the associated transmission sensitivity (green-dashed line), defined as the derivative of transmittance with respect to the logarithm of conductivity. Also marked on the graph are a typical minimum DC conductivity of graphene, 4e 2 /h ~0.15 mS (orange line), and the range of Si 2D hole gas DC conductivity (grey shaded area). Full size image After removing the substrate effects due to the cavity oscillation and the voltage-independent attenuation in the bulk p- Si substrate ( Fig. 2c ), a flat intensity modulation depth of ~16% is obtained in the 570–630 GHz frequency band. Calculated absorption, reflectance and transmittance, as a function of single-layer graphene conductivity, are presented in Fig. 2d,e , with the substrate effects removed. A striking feature shown in Fig. 2d is that absorption in single-layer graphene can be as high as 50% for terahertz beams, compared with 2.3% in the infrared/visible region. The extraordinarily large absorption implies a large number of allowed intraband transitions, which is due to the large number of available carriers and density of states in graphene, at high conductivities. Another interesting feature is that the peak absorption occurs near 5 mS due to the competing process of reflection, which reduces the number of photons that can be potentially absorbed. At very high graphene optical conductivities, transmittance approaches zero as reflectance approaches unity. Also shown in Fig. 2e is how sensitively transmittance changes with conductivity. The most significant change of transmittance occurs for the conductivity ranging from 0.1 to 50 mS with a maximum near 3 mS, which is within the tunable conductivity range of a single 2DEG or 2DHG. For instance, higher than 5 mS can be achieved in a 2DEG in AlN/GaN heterostructures [35] with n s =2×10 13 cm −2 and μ ~2,000 cm 2 V −1 s −1 , or a 2DEG/2DHG in graphene with n s =2×10 12 cm −2 and μ =20,000 cm 2 V −1 s −1 , corresponding to a DC conductivity (or sheet conductance) of 6.4 mS (or mS-square). For the range of graphene conductivity investigated in this study (pink-shaded region), the observed terahertz modulation is largely due to the change of absorption in graphene. As a result, terahertz beam absorption by single-layer graphene in this experiment is tuned from ~5 to ~20% under the bias condition used, which is remarkable because the active device is only one single-layer graphene. It is interesting to note that the minimum conductivity of graphene does not introduce appreciable terahertz insertion loss: absorption <5% (~0.2 dB) and reflection ~0 assuming a minimum conductance of 4 e 2 /h . An insertion loss of 5% is close to our experimental observation while being a conservative estimate of the graphene minimum AC conductivity [19] , [36] , based on the experimentally measured DC conductivity [37] . This means that extremely low intrinsic signal attenuation can be achieved in graphene terahertz modulators: <0.2 dB per single-layer graphene. When employing substrates with low refractive indices and/or small optical thicknesses, signal attenuation due to air/substrate reflections and cavity effects can be controlled to be <0.5 dB ( Supplementary Fig. S1 and S2 ); for instance, in a suspended graphene modulator with a total thickness of <10 μm. Although fabrication details of these envisioned graphene modulators are topics of future studies, it is worth mentioning that various large area nano-membranes have been demonstrated, for example, Constancias et al . reported silicon membranes of 100 nm thick over 3 mm×3 mm area with perfect planarity (<1 nm) [38] . Our findings are consistent with the recent reports by Horng et al . [16] and Winnerl et al . [19] , two independent studies we became aware of during the course of this manuscript preparation. Horng et al . aimed to determine the Drude weight in graphene and also observed gate-induced change of terahertz/infrared transmittance in the range of 0.9–180 THz (30–6,000 cm −1 ) using Fourier transform infrared spectroscopy, a demonstration of the underlying operating principle of the terahertz modulators investigated in our work. Winnerl et al . examined photoexcited-carrier dynamics in epitaxial graphene near the Dirac point and confirmed the validity of the simple Drude model. The study of Winnerl et al . also suggests that the nonlinear response of graphene under strong terahertz radiation may induce changes in insertion loss by graphene at Dirac point. Dynamic characteristics and broadband operation The modulation speed was measured and the results are shown in Fig. 3 . From the response waveform to a square modulation voltage, the 10–90% rise time is found to be 38 μs; thus, the 3 dB bandwidth ( f c ) is calculated to be ~18 kHz. This result matches well with the directly measured 3 dB bandwidth of ~20 kHz. To estimate the device RC time constant, a resistance ( R ) of 1,111 Ω is used, which is half of the inverse of the measured graphene conductance averaged over a V g sweep of 20–35 V. The resistance resulting from the Si substrate is neglected under this bias condition, as a 2DHG is accumulated near the Si/SiO 2 interface, and the overall resistance of the Si substrate is several orders of magnitude smaller than that of graphene. A capacitance ( C ) of 0.067 μF is calculated using a SiO 2 thickness of 95 nm and an active device (graphene) area of 1.4×1.4 cm 2 . The inverse of the calculated RC time constant corresponds to ~13 kHz, in good agreement with the directly measured modulation speed of the device. Other effects such as trap response can limit the high-speed operation of graphene-based modulators; however, for the device investigated in this study, it is reasonable to conclude that the device bandwidth is limited by its RC constant. 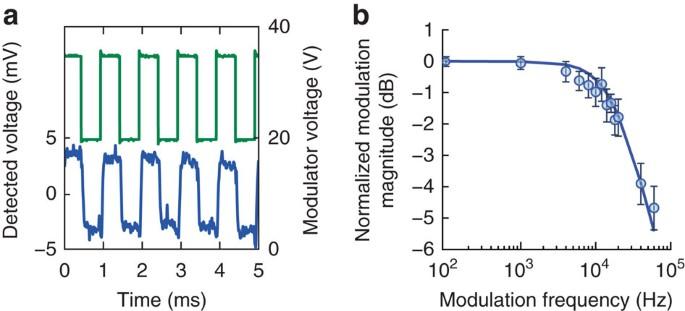Figure 3: Measured dynamic characteristics. (a) Modulator performance showing the square-wave drive voltage (green) and the modulated terahertz beam signal at the detector (blue) for a carrier frequency of 570 GHz. (b) Normalized modulation magnitude, showing a 3 dB operation bandwidth of ~20 kHz. The bandwidth is limited by the parasiticRCresponse of the device. The error bars represent the root-mean-square-deviation of the measured amplitude at each frequency. Figure 3: Measured dynamic characteristics. ( a ) Modulator performance showing the square-wave drive voltage (green) and the modulated terahertz beam signal at the detector (blue) for a carrier frequency of 570 GHz. ( b ) Normalized modulation magnitude, showing a 3 dB operation bandwidth of ~20 kHz. The bandwidth is limited by the parasitic RC response of the device. The error bars represent the root-mean-square-deviation of the measured amplitude at each frequency. Full size image In Fig. 4 , the theoretical [27] and experimental (from refs 25 , 26 and this work) intensity transmittance is plotted for several 2DEG-based terahertz modulator devices as a function of conductivity, showing a good agreement between our theory and experiments and predicting a nearly 100% modulation by single-layer graphene, using the highest experimental conductivity values reported in the literature [29] . The excellent match between the simulation and the experimental results using the DC graphene conductivity also suggests that the carrier scattering time in graphene τ is <250 fs as σ ( ω )= σ DC ( E F )/(1+ ω 2 τ 2 ). Therefore, the graphene modulator is expected to operate in a broadband range with carrier frequencies of up to at least 630 GHz, which is the highest frequency used in this experiment. The modulation efficiency in graphene will decrease with increasing frequency of the terahertz beam beyond ω ~1/ τ . The non-uniformity observed in 2D spatial transmittance maps in this study ( Supplementary Fig. S3 ) indicates that the relatively low carrier mobility (i.e. conductivity) in the large-area graphene is most likely limited by folds and breakage of graphene as well as debris resulting from the transfer process. With improved preparation of graphene leading to better uniformity and higher carrier mobility, terahertz modulation depth is expected to increase. However, the carrier-scattering-time-limited modulation bandwidth will decrease. For broadband operation, it is also necessary to eliminate the strong cavity effect by shrinking the cavity dimension along the transmission direction (substrate thickness) to be a small fraction of the terahertz beam wavelength. Our simulations show that a cavity-limited 3 dB bandwidth, as high as 9 THz, can be potentially achieved in a graphene/10-nm-Al 2 O 3 /1-μm Si device ( Supplementary Fig. S1 ). 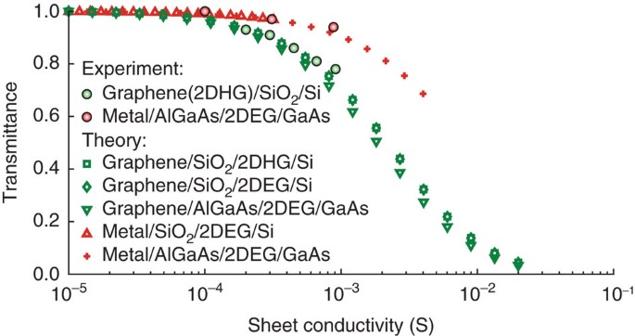Figure 4: Comparison of 2DEG-based terahertz modulators. The circles in the plot represent the experimentally observed intensity transmittance (refs25,26and this work), and the other symbols represent predicted transmittance27. Because of the adverse influence of the metal gate, modulation of terahertz transmission by tuning the 2DEG conductivity is severely reduced in the traditional 2DEG modulators27. On the other hand, by placing single-layer graphene as an active layer, instead of a gate metal, modulation can be dramatically enhanced. In the theoretical calculation, a power attenuation of 0.9 due to the metal gate was assumed; the Fermi level in graphene was set at the Dirac point at the threshold voltage of 2DEG formation in AlGaAs/GaAs or SiO2/Si heterostructures; the maximum conductivities were calculated based on the best reported values for each material system at 300 K. Figure 4: Comparison of 2DEG-based terahertz modulators. The circles in the plot represent the experimentally observed intensity transmittance (refs 25 , 26 and this work), and the other symbols represent predicted transmittance [27] . Because of the adverse influence of the metal gate, modulation of terahertz transmission by tuning the 2DEG conductivity is severely reduced in the traditional 2DEG modulators [27] . On the other hand, by placing single-layer graphene as an active layer, instead of a gate metal, modulation can be dramatically enhanced. In the theoretical calculation, a power attenuation of 0.9 due to the metal gate was assumed; the Fermi level in graphene was set at the Dirac point at the threshold voltage of 2DEG formation in AlGaAs/GaAs or SiO 2 /Si heterostructures; the maximum conductivities were calculated based on the best reported values for each material system at 300 K. Full size image By electrically tuning the density of states available for intraband transitions, transmission of terahertz waves through graphene can be controlled. On the basis of this principle, efficient broadband graphene-based terahertz modulators are proposed and experimentally demonstrated. A device prototype consisting of large area single-layer graphene on top of SiO 2 /Si was fabricated, exhibiting an intensity modulation depth of 15%, an intrinsic insertion loss of 5% and a modulation frequency of 20 kHz using a 570-GHz carrier at room temperature. To realize devices with minimum insertion loss in a broad frequency range, the substrate effects (air/substrate reflections and cavity effects) need to be minimized, which can be achieved in substrates with low refractive index and/or an optical thickness much smaller than the terahertz wavelength. Such requirements are hard to meet in the infrared/visible range (wavelength on the order of one micron); however, they are reasonably easy to satisfy in the terahertz range (wavelength on the order of hundreds of microns). Since the dynamic response of the prototype modulator is limited by the large RC time constant of the device, by reducing the device size from ~1.5 cm×1.5 cm in this study to a dimension comparable to the terahertz carrier beam wavelength, high modulation speed is expected: for instance, 2 MHz for a device of ~1.5×1.5 mm 2 (0.3 THz carrier). As high-speed graphene modulators are potentially limited by the response of slow traps in the device structure, similar to all field-effect electronic devices, they remain a topic of future studies. Owing to the facile realization and integration of the devices proposed here, graphene-based terahertz modulators seem promising for applications in several fields of terahertz technology. Sample fabrication Single-layer graphene was grown using the copper-catalysed chemical vapour deposition (CVD) approach [39] in a quartz tube furnace using CH 4 and H 2 . Following growth graphene sheets of over 1 cm 2 were transferred to host substrates (either quartz or SiO 2 / p- silicon) using Poly(methyl methacrylate) and wet-etch methods to remove the supporting metal. To study the effect of the number of graphene layers on terahertz transmission, double-layer graphene sheets were also prepared by manually stacking two sheets of single-layer CVD graphene. Shown in Fig. 5a is the graphene Raman spectrum, which was acquired with a 532-nm laser using a Witec confocal Raman microscope. High-quality single-layer graphene is confirmed by the Raman spectra as indicated by the low-intensity D peak at 1,350 cm −1 (D:G ratio ~0.2) and the characteristic 2D:G peak ratio >2. The 2D peak fits accurately to a single Lorentzian with a full width of half maximum of 33 cm −1 consistent with single-layer graphene [40] . Finally, for voltage controlled devices, top and bottom contacts were fabricated to contact graphene and p- Si, respectively. 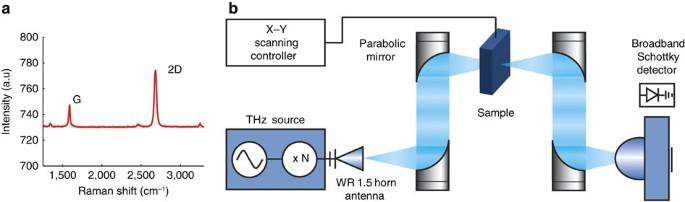Figure 5: Graphene quality and terahertz characterization set-up. (a) Representative Raman spectrum of the CVD graphene sample showing 2D:G peak ratio >2 and a weak D peak at 1,350 cm−1, characteristic of high-quality single-layer graphene. (b) Schematic of the frequency domain terahertz imaging and spectroscopy system, using a broadband Schottky diode intensity detector to measure transmission of terahertz beam in the 570–630 GHz frequency band. Figure 5: Graphene quality and terahertz characterization set-up. ( a ) Representative Raman spectrum of the CVD graphene sample showing 2D:G peak ratio >2 and a weak D peak at 1,350 cm −1 , characteristic of high-quality single-layer graphene. ( b ) Schematic of the frequency domain terahertz imaging and spectroscopy system, using a broadband Schottky diode intensity detector to measure transmission of terahertz beam in the 570–630 GHz frequency band. Full size image Terahertz modulator characterization The frequency domain terahertz transmittance measurement set-up, shown in Fig. 5b , consists of a VDI (Virginia Diodes) CW terahertz source with a tunable output in the 570–630-GHz frequency band, 4 off-axis parabolic mirrors, and a zero-bias Schottky diode broadband intensity detector [41] , [42] , [43] . The average output power of the terahertz source in this range is ~1 mW. For the terahertz signal intensity investigated in this study, the detector output voltage is linearly proportional to the detected signal power. Terahertz transmission spectroscopy was performed by sweeping the source frequency, and transmittance was calculated by normalizing the detector response with the sample to that without the sample. Data filtering was used to subtract the effect of standing waves generated in the set-up as necessary. 2D images were produced by scanning using an x – y mechanical stage, on which the sample was mounted. The imaging spatial resolution is determined by the minimum terahertz beam width of the set-up, which is estimated to be ~1.5 mm at 600 GHz. Terahertz transmittance mapped on graphene transferred on quartz showed that the transmittance for double-layer graphene is lower than that for single-layer graphene, clearly indicating that graphene is responsible for the terahertz attenuation ( Supplementary Fig. S2 ). Transmittance calculations The effect of graphene on terahertz beam transmittance has been evaluated using analytical scattering matrix as a function of graphene optical conductivity and terahertz beam frequency, for the substrate structure used in this study ( Supplementary Fig. S4 ). An air/graphene/dielectric interface is modelled with Fresnel coefficients ( S ) by treating graphene as a zero thickness conductive medium [44] : where Z 0 =376.73 Ω is the vacuum impedance, σ s is the graphene optical conductivity, and n air and n diel are the refractive index of air ( n air =1) and dielectric, respectively. For each of the other interfaces and propagation in dielectric media, classical formulas for the Fresnel coefficients are adopted [7] : where S ij stands for the scattering matrix from medium i to medium j , n i ( j ) represents the refractive index of medium i ( j ); the scattering matrix for propagation with a distance d in dielectric medium i is represented by S i,d , where k 0 =2π /λ 0 with λ 0 =c/f and c being the speed of light in vacuum. Effect of voltage-dependent conductivity in Si Further justifications are necessary for neglecting the change in Si conductivity for terahertz modulation (voltage-dependent free carrier absorption in Si). From the C–V measurement, it was found that the p -Si substrate was under depletion or weak inversion at 0 V, but a 2DHG accumulated in the p -Si substrate near the Si–SiO 2 interface at 50 V. The corresponding energy-band diagrams at 0 and 50 V are shown in the inset of Fig. 2a . Accumulation of a 2DHG indicates that when the gate voltage was swept from 0 to 50 V, the terahertz transmission through the graphene decreased, whereas that through the 2DHG in Si increased, thus the measured net transmittance modulation is smaller than that of graphene alone. The maximum amount of terahertz modulation due to the substrate can be estimated by assuming 2 sheets of charges separated by the 95 nm SiO 2 : one sheet of holes in the graphene and the other sheet of the holes at the Si substrate surface. The average low field hole mobility in graphene is calculated to be ~600 cm 2 V −1 s −1 over the voltage range of 0–50 V, and C SiO2 being the oxide capacitance. On the other hand, the mobility of 2D holes in Si is on the order of 80 cm 2 V −1 s −1 for a concentration of n 2DHG = C SiO2 ΔV g / e =1×10 13 cm −2 , which is the maximum 2DHG concentration possible under accumulation [45] . As a result, the conductivity modulation in the Si 2DHG is at least 7.5 times smaller than that of graphene. Taking into consideration the modulation due to the 2DHG in Si, the intensity modulation of terahertz beams due to graphene alone is therefore 15±2%. How to cite this article: Sensale-Rodriguez, B. et al . Broadband graphene terahertz modulators enabled by intraband transitions. Nat. Commun. 3:780 doi: 10.1038/ncomms1787 (2012).